A self-propelled biohybrid swimmer at low Reynolds number Many microorganisms, including spermatozoa and forms of bacteria, oscillate or twist a hair-like flagella to swim. At this small scale, where locomotion is challenged by large viscous drag, organisms must generate time-irreversible deformations of their flagella to produce thrust. To date, there is no demonstration of a self propelled, synthetic flagellar swimmer operating at low Reynolds number. Here we report a microscale, biohybrid swimmer enabled by a unique fabrication process and a supporting slender-body hydrodynamics model. The swimmer consists of a polydimethylsiloxane filament with a short, rigid head and a long, slender tail on which cardiomyocytes are selectively cultured. The cardiomyocytes contract and deform the filament to propel the swimmer at 5–10 μm s −1 , consistent with model predictions. We then demonstrate a two-tailed swimmer swimming at 81 μm s −1 . This small-scale, elementary biohybrid swimmer can serve as a platform for more complex biological machines. Many biological species, including bacteria, protozoa and spermatozoa, use flagella to swim in complex fluids [1] . These swimmers function at small characteristic length scales in the low Reynolds number ( Re ) regime, where viscous forces dominate inertial forces. To generate propulsion at this scale, the swimmers must produce a time-irreversible deformation of the flagella [2] . Spermatozoa, for example, generate complex bending patterns in their flagella by sliding microtubules relative to each other [3] , [4] , [5] , whereas bacteria rotate helix-shaped flagella to generate propulsion [6] . Although such low Re swimmers are ubiquitous in nature, there have been only a few experimental realizations of flagellar propulsion using synthetic materials, all of which rely on external magnetic drivers. These include a magnetic cork-screw swimmer [7] , [8] and a flagellar swimmer formed by a string of magnetic beads connected by DNA molecules [9] . These swimmers are twisted or deflected by an external oscillatory magnetic field to generate propulsive thrust. In addition, bacteria and spermatozoa have been used to propel microspheres and other microfabricated structures, relying on the natural propulsive mechanism of the driving flagella [10] , [11] . To date, there is no demonstration of a self propelled, synthetic flagellar swimmer operating at low Re , despite potential applications in the in vivo or in vitro transport and delivery of cargo. Accompanied by required advances in the construction of cellular circuits, such a swimmer could respond to external stimulation, such as gradients in chemistry, temperature and light, and autonomously navigate in a complex fluidic environment. Here we demonstrate a functional motile platform that can be further developed into such a biohybrid machine. To produce microscale flagellar propulsion, we must address two significant hurdles. First, for independent swimming, the swimmer must either be flexible or have moving joints. Second, a suitably scaled driving mechanism must be integrated with the synthetic flagellum to produce the required deformation force. Here we utilize a novel fabrication process [12] to produce highly compliant polydimethylsiloxane (PDMS) filaments on which we directly culture contractile cells. We use a slender-body hydrodynamics model to design the flagella such that given proper placement of contractile cells, forward swimming is achieved. The resultant one-dimensional swimmer mimics the structure of the spermatozoon ( Fig. 1a ), consisting of a long, slender tail and a short, rigid head, with cardiomyocytes selectively cultured on the tail. Periodic contractions of the cardiomyocytes generate a bending wave that propagates from the actuation site to the free end of the tail, producing a net thrust that propels the swimmer forward. 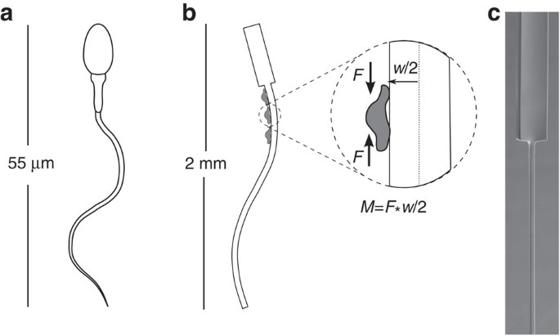Figure 1: Concept design of a biohybrid flagellum. (a) Spermatozoa swim at lowRenumber by generating complex time-irreversible waveforms throughout a long, slender tail. (b) Proposed biohybrid swimmer, consisting of an elastic filament with a rigid head and a compliant tail, and a small, single cluster of contractile cells generating a forceFat a distancew/2 from the filament’s neutral axis. (c) Scanning electron micrograph of a fabricated PDMS filament near the head/tail junction. The head and tail are 57 and 7 μm wide, respectively, and 22 μm deep. Figure 1: Concept design of a biohybrid flagellum. ( a ) Spermatozoa swim at low Re number by generating complex time-irreversible waveforms throughout a long, slender tail. ( b ) Proposed biohybrid swimmer, consisting of an elastic filament with a rigid head and a compliant tail, and a small, single cluster of contractile cells generating a force F at a distance w /2 from the filament’s neutral axis. ( c ) Scanning electron micrograph of a fabricated PDMS filament near the head/tail junction. The head and tail are 57 and 7 μm wide, respectively, and 22 μm deep. Full size image Determination of swimmer parameters The location of the cardiomyocytes determines the swimming dynamics. If cardiomyocytes were uniformly cultured on the entire filament, synchronous beating of the cells [13] would cause simultaneous bending and relaxation of the filament along its length, yielding a time-reversible deformation and zero net motion, reminiscent of the scallop theorem [2] . To achieve time irreversibility, cells are selectively seeded on a single region of the filament, leaving the remainder of the filament to deform passively in response to fluid drag ( Fig. 1b ). The resultant mechanism is functionally different from that of the spermatozoon, which is capable of generating force throughout its flagellum. By appropriate selection of the actuating location, forward or backwards propulsion is realized. Thus, we create a microscale swimmer that propels itself by transforming the contractions of cardiomyocytes in situ into time-irreversible deformations of the filament. Cardiomyocytes generate 1–10 μN force [14] . Populations of cardiomyocytes have been used as actuators in a variety of macroscopic mechanical devices that operate at high Re , including a millimetre-scale pump [15] , autonomous or paced walkers or swimmers [16] , [17] , and a jellyfish [18] , all involving two-dimensional films or three-dimensional structures. These larger scale devices, with millimetre to centimetre scale deformations, generate propulsion by high Re mechanisms that are not viable at the microscale. To create a microscale swimmer capable of being driven by one to several cardiomyocytes at low Re , an appropriate filament compliance must be selected such that the filament can be deflected by cell contractions, and yet is sufficiently rigid to maintain its shape under the application of static contractile cell forces. For our swimmers, rectangular cross-sections ( Fig. 1c ) with a high (3:1) aspect ratio are chosen so that the top and bottom surfaces are too narrow for cell adhesion, limiting cell attachment to the sides of the filament. The depth is just sufficient for cells to attach and generate contractile forces along the longitudinal direction. Such geometric confinement has been shown to induce sarcomeric alignment in cardiomyocytes [19] . For our case, this alignment serves to maximize contractile force in the desired direction. The contraction of the cardiomyocytes creates a bending moment about an axis orthogonal to the page in Fig. 1b , confining the filament deformation to a single plane (the plane of the paper in Fig. 1b ). After conducting several experiments, we find that a filament depth of 20–30 μm and a filament width of 7–10 μm satisfy these requirements. The remaining dimensions of the swimmer, the cross-section of the head and the lengths of the head and the tail, critically affect swimming dynamics. A rigid head is chosen to optimize swimmer performance, as any bending of the head would generate a propulsive force opposite to that generated by the tail. We design heads with a width of 30–70 μm to provide a sharp increase in stiffness over the tail. In addition, the length of the head relative to the tail influences the amplitude of the propagating wave in the tail. A very long head would maximize the amplitude of the tail deflection, increasing propulsion. However, this would come at the cost of a large longitudinal drag, thus compromising the swimming speed. A very short head, on the other hand, would rotate with large amplitude, resulting in minimal tail deflection and little generated propulsive force. To select the lengths of the head and the tail, we model the swimmer as a slender-body elastohydrodynamic system based on previously established theory [1] , [20] , [21] , [22] , [23] . We consider a free filament driven by an onboard periodic actuator. Placing the x axis along the relaxed filament, with the origin at the front of the swimmer head, and selecting the y axis such that filament deformation lies in the x–y plane ( Fig. 2a ), we balance all forces normal to the filament [20] while assuming small angle displacements (| y x |<<1). With subscripts denoting partial differentiation, fluid drag generates a force of f D =−ζ ⊥ y t and the bending of an elastic filament generates a restorative force of f E =− Ay xxxx , both per unit length of the filament. Here, ζ ⊥ is the normal drag coefficient and A is the filament stiffness computed as the product of elastic modulus E and area moment of inertia I . ζ ⊥ and A are treated as position-varying parameters to account for the increased width of the head. The system is driven by a bending moment applied at the location on which cells are cultured, and has time dynamics and magnitude estimated from experimental observation ( Fig. 2b ). 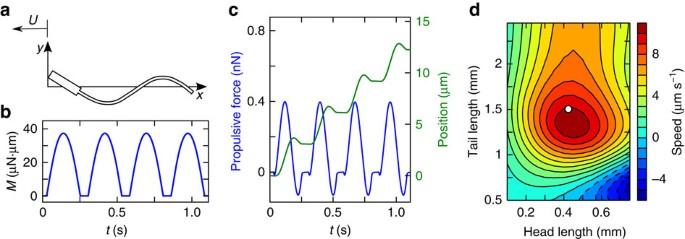Figure 2:Prediction of swimming by the model represented byequation1. (a) Local coordinate system for analysis of swimmer. (b) Driving moment applied over a span of 60 μm adjacent to head/tail junction. (c) Resultant propulsive force (blue) and swimmer position (green) as function of time, for a filament with a 424-μm-long head and a 1,503-μm-long tail, and a max applied moment of 38 μN·μm (Supplementary Movie 1). Positive positions and forces correspond to swimming towards the head. (d) Map of predicted velocity (colorbar) as a function of head length (xaxis) and tail length (yaxis). The white dot corresponds to the dimensions of the swimmer inFig. 4. This bending moment M ( x , t ) is equivalent to a normal force f C = M xx ( x , t ), providing the final term of the governing equation: Figure 2: Prediction of swimming by the model represented by equation 1 . ( a ) Local coordinate system for analysis of swimmer. ( b ) Driving moment applied over a span of 60 μm adjacent to head/tail junction. ( c ) Resultant propulsive force (blue) and swimmer position (green) as function of time, for a filament with a 424-μm-long head and a 1,503-μm-long tail, and a max applied moment of 38 μN·μm ( Supplementary Movie 1 ). Positive positions and forces correspond to swimming towards the head. ( d ) Map of predicted velocity (colorbar) as a function of head length ( x axis) and tail length ( y axis). The white dot corresponds to the dimensions of the swimmer in Fig. 4 . Full size image The ends of a filament of length L are free from any forces (torque or shear), resulting in the free boundary conditions y xx (0)= y xxx (0)= y xx ( L )= y xxx ( L )=0. This ensures zero net torque and transverse forces on the swimmer, resulting in zero net translation along the y axis or in-plane rotation. We solve equation 1 for y ( x , t ) ( Supplementary Fig. 1 and Supplementary Movie 1 ) via a finite difference method, and then calculate the propulsive force F p ( t ) by projecting the fluid drag reaction force on the x axis ( Fig. 2c ): F p ( t )= ζ ⊥ −ζ ∥ ) y t y x dx . Here, ζ ∥ is the tangential drag coefficient which varies with x along with ζ ⊥ to account for variation in filament cross-section. The net filament velocity u in the x direction is determined by balancing the tangential drag with the propulsive force: u ( t )= F p ( t )/( ζ ∥ ( x ) dx ). To determine optimal filament parameters, we plot the mean velocity for a range of head and tail lengths ( Fig. 2d ). A maximum swimming velocity is predicted for head and tail lengths of 450 and 1,350 μm, respectively, providing a target for the swimmer parameters. Elastohydrodynamic systems are often characterized by the dimensionless Sperm number [9] , defined as S p = L / , where ω is the displacement frequency of the filament. For head lengths L H between 200 and 500 μm, numerical solutions predict maximum swimming velocities for S p between 3.5 and 4 ( Supplementary Fig. 2 ). We fabricate long, thin PDMS filaments ( Fig. 1c ) with precise control over filament dimensions by filling a microfabricated channel with liquid PDMS using capillary draw [12] (see Methods). We selectively seed cardiomyocytes on a preselected region of the PDMS filament to restrict the actuation to a specific location. Selective seeding is achieved by functionalizing the filament near the head region with an extracellular matrix for cell adhesion (see Methods). The rest of the tail is coated with a cell de-adherent, limiting cell adhesion to the desired region. The cardiomyocytes generate contractile forces on the filament surface, at a distance of half the filament width from its neutral axis, resulting in a bending moment and angular deflections of 30–45° ( Fig. 3 and Supplementary Movie 2 ). The swimmer is maintained in culture media at 37 °C and 5% CO 2 . Although this is a significant functional limitation, an alternative cell type, such as turtle cardiomyocytes, could be selected to facilitate functionality at room temperature and in anoxic environments [24] . 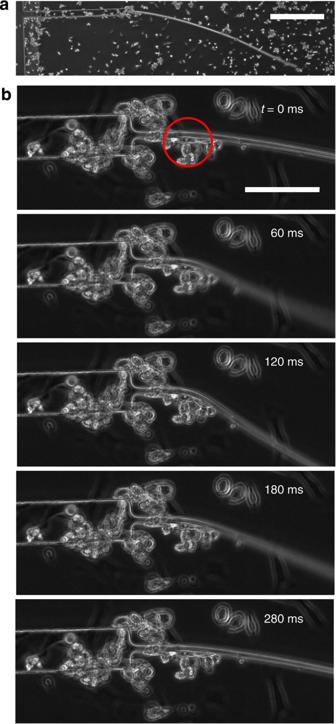Figure 3: One-dimensional filament actuated by cardiomyocyte contractions. (a) PDMS filament 48 h after cell culture, with head still fixed to substrate and tail cut free and detached from substrate. Cardiomyocytes are allowed to attach near the head region of the filament only. Scale bar, 400 μm. (b) Close-up image of the head region showing the contractile cells (circled in red) and the corresponding deformations of the filament during a complete cycle. The maximum moment estimated from the elastic bending of the filament is 38 μN·μm with a frequency of ~3 Hz (Supplementary Movie 2). Scale bar, 100 μm. Figure 3: One-dimensional filament actuated by cardiomyocyte contractions. ( a ) PDMS filament 48 h after cell culture, with head still fixed to substrate and tail cut free and detached from substrate. Cardiomyocytes are allowed to attach near the head region of the filament only. Scale bar, 400 μm. ( b ) Close-up image of the head region showing the contractile cells (circled in red) and the corresponding deformations of the filament during a complete cycle. The maximum moment estimated from the elastic bending of the filament is 38 μN·μm with a frequency of ~3 Hz ( Supplementary Movie 2 ). Scale bar, 100 μm. Full size image Experiment Guided by the theoretical model, we fabricate the biohybrid swimmers. 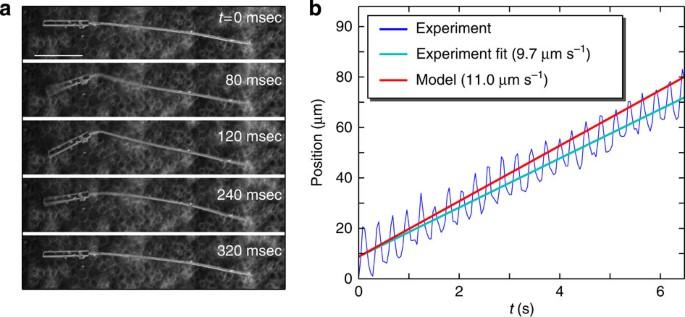Figure 4: Experimental realization of a free-swimming biohybrid filament. (a) Sequence of filament displacement shapes over a complete cycle during swimming (Supplementary Movie 4). Scale bar, 400 μm. (b) Resultant displacement with time along the filament direction (blue), with a mean velocity of 9.7 μm s−1(light blue), compared with the model prediction of 11.0 μm s−1(red). Figure 4a presents a specimen with a 424-μm-long head and 1,503-μm-long tail. Primary cardiomyocytes and fibroblasts from neonatal rats are seeded on the entire swimmer. Cells attach only to the head and the part of the tail immediately adjacent to the head due to selective functionalization ( Fig. 3 and Supplementary Movies 2 and 3 ) and form a cluster occupying a length of 60–100 μm of the filament. On the basis of the size of the cardiomyocytes, we estimate that the cluster contains one to three cardiomyocytes. Two to three days after seeding, the swimmer is released into suspension in a petri dish on a thin layer of Percoll, a biocompatible solution of silica nanoparticles. PDMS is lighter than Percoll but heavier than cell culture media. Hence, the swimmer floats at the interface between Percoll media and normal media ~1 mm above the floor, where the wall effects from fluid interaction with the substrate are minimal [25] , [26] . Confining the motion of the swimmer to a horizontal plane is essential for imaging and subsequent analysis. Cells on the filament contract with a frequency of ~3 Hz and the biohybrid structure swims forward at a velocity of 9.7 μm s −1 ( Fig. 4b and Supplementary Movie 4 ). The swimmer tends to roll slowly about the axis of the relaxed filament, at approximately one full rotation per minute. This is likely to be due to a slight out-of-plane component of the filament deflection producing a small torque about the axis of the filament. To test the potential lifespan of the swimmers, we culture cardiomyocytes on a set of swimmers, free the tail, but leave the head anchored to the substrate. We find that the filaments are capable of beating for 3–4 days ( Supplementary Fig. 3 ), suggesting a similar potential lifespan for free swimmers. However, the lifetime of free swimmers could not be properly evaluated, as they either get stuck to the wall of the petri dish or are washed out during cell media changes before contractility ceased. Figure 4: Experimental realization of a free-swimming biohybrid filament. ( a ) Sequence of filament displacement shapes over a complete cycle during swimming ( Supplementary Movie 4 ). Scale bar, 400 μm. ( b ) Resultant displacement with time along the filament direction (blue), with a mean velocity of 9.7 μm s −1 (light blue), compared with the model prediction of 11.0 μm s −1 (red). Full size image We compare the observed swimming dynamics with those predicted by the computational model by using the physical parameters of the swimmer, that is, swimmer geometery, elastic modulus, drag coefficients and driving moment magnitude and location. The maximum cell-generated moment and driving frequency are estimated from the maximum observed filament curvature and its periodicity during swimming. The normal drag coefficient ζ ⊥ for the tail is measured to be 9.25 mPa·s (see Methods) by holding the swimmer in a uniform flow field and measuring the tail deflection produced by fluid drag. ζ ∥ is estimated by the approximation ζ ⊥ ≈2ζ ∥ (ref. 1 ), which is expected to overestimate propulsion for a filament of finite width [27] . The model predicts a mean swimming velocity of 11.0 μm s −1 , close to the observed speed of 9.7 μm s −1 ( Fig. 4b ). For this swimmer, we calculate the Reynolds number as Re = =1.8 × 10 −2 , where μ is the fluid viscosity and ρ is the fluid density, consistent with the model assumption. The sperm number, S p =4.19, is close to the optimum to maximize speed. 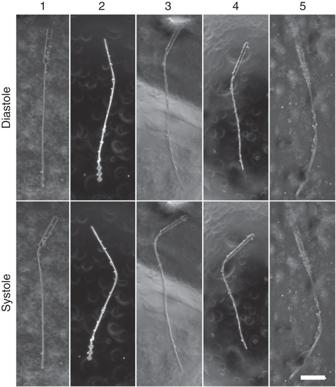Figure 5: Additional single-tailed swimmers. Five sample swimmers in systole and diastole (see alsoSupplementary Movie 5), exhibiting swimming velocities of 9.7, 4.0, 5.8, 4.6 and 3.8 μm s−1, respectively. Characteristic metrics for each swimmer, including model predictions, are tabulated inSupplementary Table 1. Scale bar, 300 μm. Figure 5 contains micrographs of the sample in Fig. 4 and four additional swimmers in the systolic and diastolic phases. These swimmers exhibit swimming velocities between 3.8 and 9.7 μm s −1 . Supplementary Fig. 4 and Supplementary Table 1 provide relevant parameters for each swimmer, including model predictions, showing the effect of variability in cell plating, cell force and contractile frequency on swimming speeds. Although we have control over filament cross-sections and locations of cell actuation, there is intrinsic variation in the dynamics of actuating cardiomyocytes. The five samples in Fig. 5 , for example, exhibit estimated peak contractile forces of 4.4–14.4 μN, with contractile frequencies of 1.6–3.6 Hz. Figure 5: Additional single-tailed swimmers. Five sample swimmers in systole and diastole (see also Supplementary Movie 5 ), exhibiting swimming velocities of 9.7, 4.0, 5.8, 4.6 and 3.8 μm s −1 , respectively. Characteristic metrics for each swimmer, including model predictions, are tabulated in Supplementary Table 1 . Scale bar, 300 μm. Full size image By functioning in a turbulence-free, low Re environment, we are able to predict swimming dynamics with a high degree of accuracy. In essence, each contraction of the driving cells causes the swimmer to take a single step forward through the suspending fluid. This makes the system suitable for integrating into more complex arrangements to achieve diverse functionality. For example, the model predicts that the direction of swimming depends on the location of the actuation site along the filament ( Supplementary Fig. 5 ). Here we consider a homogenous filament without a head. For actuation anywhere but the middle of the filament, non-zero net propulsion is predicted, with resultant swimming in the direction of the filament half containing the actuator. To verify this prediction, we seed cells near the end of the tail of a filament. The swimmer now swims backwards ( Supplementary Fig. 6 ). This suggests the potential for creating a filament with multiple, discrete actuation sites, providing a mechanism for controlling directionality of the swimmer. All demonstrated single-tailed swimmers exhibit low swimming velocities, travelling ~10 −3 their body length per second. Each of these swimmers utilizes a head that swings through the fluid to provide a counteracting moment to balance the moment produced by the motion of the tail. This swinging head is a significant energy drain. In Fig. 6 , we present a two-tailed swimmer consisting of a pair of synchronized actuators on a homogenous filament. The simultaneous contraction of these actuators causes the deflection of a pair of propulsion generating filaments, eliminating the need for a head to provide moment balance. Synchronized actuation of the pair of filaments is critical for optimal functionality and can be achieved by electrical coupling of contractile cells through gap junctions. This configuration generates significantly higher propulsion, attributed to the additive effect of multiple force generating filaments, the effective fixed boundary condition at the base of each filament provided by this moment-balancing design, and the reduced longitudinal drag associated with the shorter length of this configuration. These effects, combined, yield a measured swimming velocity of 81 μm s −1 , or 8.3% its body length per second, a vast improvement over single-tailed samples. Model predictions are unavailable for this case due to significant deviation from the assumed small-angle form of the single-tailed swimmers. This swimmer provides an example of how elementary one-tailed swimmers can be combined to achieve significantly higher speeds. 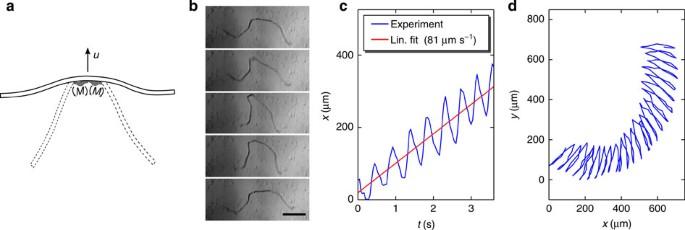Figure 6: Two-tailed swimmer. (a) Schematic of two-tailed swimmer, with a pair of actuation sites producing momentMand driving a pair of tails. (b) Sequence of actuation of two-tailed swimmer. Scale bar, 400 μm. (c) As no passive head is required to provide a moment balance around the actuation point, all fluid drag contributes to the passive deformation of the filaments and the generation of propulsive force, permitting significantly higher swimmer velocities (linear fit: 81 μm s−1), with correspondingRe=0.14. (d) The right-hand tail provides more propulsive force than the left, causing the swimmer to move in an anticlockwise circular pattern (seeSupplementary Movie 6). Figure 6: Two-tailed swimmer. ( a ) Schematic of two-tailed swimmer, with a pair of actuation sites producing moment M and driving a pair of tails. ( b ) Sequence of actuation of two-tailed swimmer. Scale bar, 400 μm. ( c ) As no passive head is required to provide a moment balance around the actuation point, all fluid drag contributes to the passive deformation of the filaments and the generation of propulsive force, permitting significantly higher swimmer velocities (linear fit: 81 μm s −1 ), with corresponding Re =0.14. ( d ) The right-hand tail provides more propulsive force than the left, causing the swimmer to move in an anticlockwise circular pattern (see Supplementary Movie 6 ). Full size image In this work we demonstrate the feasibility of an elementary flagellar swimmer actuated by contractile cells. We analyse the swimmer with a computational model to provide a basis for parameter selection. For swimmers exhibiting low-angle filament displacements, the model provides accurate results. It is a general model based on slender body, low- Re hydrodynamics that predicts the dynamics of a swimmer consisting of a tail, with or without a head. The model accounts for arbitrary filament material properties, geometries and drag coefficients. It permits the application of an arbitrary actuation as a function of time and location along the tail. To model a specific swimmer, we measure these parameters and use them as inputs for the model to predict the resultant swimming dynamics. All model parameters are determined independently of the observation of the free swimmer with the exception of amplitude and frequency of contractile force and the exact location of the contractile cells. These parameters exhibit significant variation between experiments with notable effect on the resultant swimming dynamics. Supplementary Table 1 tabulates these effects for five swimmers where Re varies between 10 −3 and 10 −2 , and S p varies between 2 and 5. Deviations in the model predictions from observed swimming speeds are attributed to error in the measurement of these parameters. Such measurements can be improved by, for example, measuring filament cross-sections using scanning electron microscopy. Our swimmer speeds scaled by their overall length are notably slower than their biological counterparts. For example, the bull spermatozoon, with a 70-μm length, swims at 97 μm s −1 , or 139% of its body length per second [28] , whereas our single-tailed and two-tailed swimmers manage velocities of just 0.5% and 8.3% their body length per second, respectively. The improved performance of the bull spermatozoon is enabled by its shorter length, higher frequency actuations, higher angular amplitude actuations and the capacity to continuously deform the flagella along its length to provide complex shapes to maximize propulsion. Our swimmers are limited to a single point of actuation, relying on passive deformation of the filament to provide thrust. Contractile frequency is dictated by the selection of cells and environmental conditions. For the demonstrated filament widths, our computational model indicates that our parameter selection is nearly optimal ( Fig. 2d ). As such, we must look to other mechanisms to improve performance. We have already demonstrated an order-of-magnitude improvement in scaled swimming velocity with a two-tailed design, which could be scaled up with appropriate fabrication techniques. Furthermore, additional tails also provide the capacity for navigation. Although single-tailed biological species can turn by generating appropriate complex flagellar deformations, our demonstrated filament deformations are constrained to a single shape determined by contractile strength and frequency. If multiple tails can be combined with cells that selectively contract based on a suitable control mechanism, the propulsive force applied at different locations of the swimmer can be modulated to provide asymmetry and resultant steering. As proof of concept, the two-tailed swimmer ( Fig. 6 and Supplementary Movie 6 ) generates a slight imbalance in the propulsion generated by each tail, resulting in a curved swimmer trajectory. Extending this mechanism to three or more tails and employing neurons and muscle cells to selectively actuate individual filaments could enable a swimmer capable of navigation in three-dimensions with on-board control. For the 7- to 10-μm width filaments presented in this manuscript, the tail length must be on the order of the characteristic length ≈1 mm. Thus, to improve scaled swimmer velocity by shortening our swimmer length, we would have to simultaneously reduce the filament radius (filament stiffness A r 4 ). We have reduced the filament width to 4–5 μm and, with further process refinements, expect to reduce them to within 1 μm, reducing the optimal filament length to ~100 μm. However, for this design to function, a variable-width swimmer would be required, as culturing cardiomyocytes directly on such a thin tail would yield uncontrollable curls and twists due to the static contractile force generated by the cells. Thus, an intermediate width would be required for the actuation location that tapers down to the passive, propulsion generating region. However, the size of the eukaryotic cells powering our swimmers provides a lower bound to potential total swimmer size, making it infeasible to reduce our total length to the size of a mammalian spermatozoon or the previously demonstrated 1–2 μm magnetic swimmers [9] . Our microscale filaments provide a unique platform to probe the two-way interaction between contractile cells and their substrate. Supplementary Movie 7 depicts the long-term interaction between cardiomyocytes cultured on a thin PDMS filament. Over several days, cells generate increasing static contractile forces, producing large-scale bending deformations of the filament. These deformations increase the effective moment arm of the cells by increasing their distance from the filament neutral axis. This effectively increases filament compliance, thus allowing increased bending in response to periodic contractions. Such a nonlinear dynamic feedback between the cells and the substrate may yield the emergence of cell clusters with specific functionality and architecture, warranting further fundamental biological studies. The characterization and exploitation of such nonlinear interactions may facilitate the development of more complex biological machines. To summarize, we demonstrate a biohybrid flagellar swimmer propelled by contractile cells that operates at low Re . We provide the necessary theoretical framework to design such swimmers and to accurately predict their performance. Our method of making the swimmer is amenable to batch fabrication, as it is based on standard lithographic techniques and mass-scale cell plating. Although only cardiomyocytes are used as contractile cells in this work, the method is applicable to other homotypic cell types, such as optogenetic muscle cells for light-actuated swimming, or heterotypic cells types, such as turtle cardiomyocytes and fibroblasts for room temperature swimming, and neurons and muscle cells for sensing-based intelligent swimming. The study thus provides a foundation for a new class of self-propelled, batch-fabricable, soft biological swimming machines. Swimmer fabrication and preparation The PDMS filament is fabricated by filling a channel in a silicon wafer with liquid PDMS by capillary draw [12] . The channel is carved by dry etching (inductively coupled plasma deep reactive-ion etching) of silicon to the desired depth of the filament and coating the wafer with a thin layer of polytetrafluoroethylene to reduce stiction with the cured PDMS filament ( Fig. 7a–d ). The cross-section of the channel determines the shape of the PDMS filament. We chose a rectangular cross-section for developing the swimmer ( Fig. 7e ), but for demonstration we present a semicircular cross-section in Supplementary Fig. 7 . An approximately 3 mm square is etched at either end of the channel to act as a reservoir for filling the channel. PDMS (Sylgard 184, 4:1 base to crosslinker ratio) is added to each reservoir and the channel is filled by capillary draw in about 2 min. The samples are cured at 60 °C for 12 h, then inundated with ethanol, which swells the cured PDMS to facilitate the release of the filament from the channel. The filaments and square reservoirs are released manually, transferred to a 35-mm petri dish and rinsed in PBS ( Fig. 7f ). 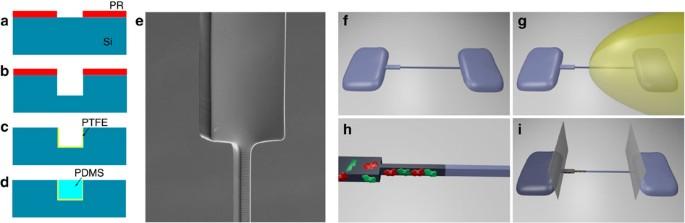Figure 7: Fabrication and selective functionalization of the PDMS filament. (a–d) Etching of silicon (Si) wafer by standard photolithography and dry etching (inductively coupled plasma deep reactive-ion etching), where PR is photoresist and PTFE is polytetrafluoroethylene. Atd, the channel is filled with liquid PDMS by capillary draw, followed by curing at 60 °C. (e) The filament is peeled from the substrate, yielding a rectangular cross-section. Non-rectangular cross-sections can be produced by isotropic etching (Supplementary Fig. 7) (f) Filament is transferred to PDMS substrate. (g) Regions where no cell adhesion is desired are masked in gelatin, and the system is incubated in fibronectin. The mask is removed and the system is incubated in Pluronic F127 (cell deadherent) and transferred to a fresh PDMS substrate. (h) Primary cardiomyocytes and fibroblasts are cultured on the filament, displaying preferential adhesion to the functionalized regions. (i) The tail is cut and peeled 24 h after culturing cells (right vertical plane), and the head is cut 48–72 h after culturing cells (left vertical plane). Figure 7: Fabrication and selective functionalization of the PDMS filament. ( a – d ) Etching of silicon (Si) wafer by standard photolithography and dry etching (inductively coupled plasma deep reactive-ion etching), where PR is photoresist and PTFE is polytetrafluoroethylene. At d , the channel is filled with liquid PDMS by capillary draw, followed by curing at 60 °C. ( e ) The filament is peeled from the substrate, yielding a rectangular cross-section. Non-rectangular cross-sections can be produced by isotropic etching ( Supplementary Fig. 7 ) ( f ) Filament is transferred to PDMS substrate. ( g ) Regions where no cell adhesion is desired are masked in gelatin, and the system is incubated in fibronectin. The mask is removed and the system is incubated in Pluronic F127 (cell deadherent) and transferred to a fresh PDMS substrate. ( h ) Primary cardiomyocytes and fibroblasts are cultured on the filament, displaying preferential adhesion to the functionalized regions. ( i ) The tail is cut and peeled 24 h after culturing cells (right vertical plane), and the head is cut 48–72 h after culturing cells (left vertical plane). Full size image To selectively functionalize the filaments and limit cell adhesion to near the head of the swimmer, a gelatin mask (from bovine, Sigma-Aldrich, 10% in PBS) is placed over regions where no cell adhesion is desired ( Fig. 7g ). The masked sample is incubated in fibronectin (BD Bioscience, 25 μg ml −1 ) at room temperature for 90 min. The samples are rinsed three times with PBS after removing the gelatin mask, then incubated for 20 min in F127 (1% in PBS, Sigma-Aldrich) to further reduce cell adhesion to the previously masked region of the filament. The device is rinsed three times with PBS and moved to a fresh PDMS substrate that has also been modified with F127 to prevent cell adhesion. Cell culture Primary cardiomyocytes are extracted from 2- to 4-day-old Sprague–Dawley rats [16] under approved Institutional Animal Care and Use Committee protocol number 11160. The hearts are immediately transferred to ice-cold Hank’s balanced salt solution after dissection. The hearts are minced into 1 mm cube sections, then digested in 0.05% Trypsin (Worthington Biochemical) at 4 °C on a shaker. After 16 h, the tissue is transferred to fresh culture media (high glucose DMEM, 2 mM L -glutamine, 10 mM HEPES, 10% fetal bovine serum and 1% penicillin–streptomycin), warmed to 37 °C and rinsed twice in Hank’s balanced salt solution. The tissue is incubated in 0.1% (w/v) type II collagenase (Worthington Biochemical) for 45 min at 37 °C. The tissues are triturated to mechanically dissociate the cells, filtered through a 75-μm cell strainer, centrifuged at 150 g for 5 min and resuspended in fresh culture media. The cells are then seeded on the functionalized filaments at a density of ~250,000 cells cm −2 ( Fig. 7h ). We find that the cardiomyocytes generate significantly higher contractility when permitted to develop on a tail that is detached from the substrate. To accomodate, we change the media after 24 h, cut the tail and peel it off the substrate, allowing cell contractions to freely deform the filament ( Supplementary Movie 3 ). Twenty-four to forty-eight hours after cutting the tail, the head is cut and the swimmer is released into suspension. To facilitate imaging and avoid sedimentation of the swimmers, ~1 ml of increased density media (50% double concentration DMEM, 50% Percoll) is added to the 35-mm petri dish. This mixed media has a measured viscosity of 1.15 mPa·s, compared with 0.82 mPa·s for plain culture media at 37 °C, measured on a temperature-controlled rheometer (TA Instruments Discovery HR-3). This increased viscosity is taken into consideration in the computational model. Measurement of parameters The elastic modulus of PDMS (4:1 base to crosslinker ratio) is measured to be 3.86 MPa by nanoindentation. The contractile force is estimated as the force required by classical beam theory to achieve the maximum observed angular deflection of the filament. This neglects the influence of the fluid drag on parts of the tail that are still in motion at the time of maximum deflection of the filament and, thus, slightly underpredicts the contractile force. The applied force, as well as the driving frequency, must be measured for each experiment to compare model results, whereas all other parameters are independently measured. The normal drag coefficient ζ ⊥ for the tail is measured experimentally by suspending a sample filament 1.5 mm above the substrate, immersed in culture media, in a petri dish. Twenty-micrometre polystyrene beads are added and a flow is induced perpendicular to the filament orientation. A velocity distribution across the tail is determined by particle tracking the suspended polystyrene beads. The drag coefficient is extracted by measuring the bending of the filament in response to fluid drag and determining the required drag coefficient to produce the observed deflection. ζ ⊥ for the head is calculated by extrapolating the measurement for the tail using the slender body theory formula for circular cross-sections ζ ⊥ = , where μ is the fluid viscosity, L is the filament length and r is the radius of the filament [1] . How to cite this article: Williams, B. J. et al. A self-propelled biohybrid swimmer at low Reynolds number. Nat. Commun. 5:3081 doi: 10.1038/ncomms4081 (2014).